Multiple recent horizontal transfers of a large genomic region in cheese making fungi While the extent and impact of horizontal transfers in prokaryotes are widely acknowledged, their importance to the eukaryotic kingdom is unclear and thought by many to be anecdotal. Here we report multiple recent transfers of a huge genomic island between Penicillium spp. found in the food environment. Sequencing of the two leading filamentous fungi used in cheese making, P. roqueforti and P. camemberti , and comparison with the penicillin producer P. rubens reveals a 575 kb long genomic island in P. roqueforti —called Wallaby —present as identical fragments at non-homologous loci in P. camemberti and P. rubens . Wallaby is detected in Penicillium collections exclusively in strains from food environments. Wallaby encompasses about 250 predicted genes, some of which are probably involved in competition with microorganisms. The occurrence of multiple recent eukaryotic transfers in the food environment provides strong evidence for the importance of this understudied and probably underestimated phenomenon in eukaryotes. Humans have created many novel, nutrient-rich and homogeneous environments exerting strong selection pressures and inducing the rapid adaptation of microorganisms, such as fungal pathogens of crops, food spoilers and domesticated fungi used for fermentation in beverage or food (for example, Saccharomyces for bread, beer and wine, Aspergillus for traditional fermented Asian foods, such as sake, soy sauce and miso, and Penicillium for cheese and cured or fermented meat). These rapid adaptations in fungi provide excellent models for studying general processes of eukaryotic genome evolution, including the functional and ecological impact of horizontal gene transfer [1] and changes in metabolism [2] . Prokaryote-to-prokaryote transfers have been recognized as common and their associated impact important enough to raise questions about the possibility of reconstructing prokaryotic history through a tree of life or to change practices relating to antibiotic use in medicine. By contrast, horizontal transfers in eukaryotic species are still perceived by many to be isolated, sporadic events with a limited impact [3] , [4] , [5] . However, over the last 20 years or so, a number of cases of gene transfer in eukaryotes have been described. These documented cases include transfers of genetic material of prokaryotic origin into a eukaryote host [6] and transfers in man-made environments, for example, between yeasts used for wine fermentation [1] or pathogenic fungi on crops [6] , [7] , [8] , [9] . Both the sizes and number of genes involved vary widely. Transfers of a single gene, a complete metabolic pathway [10] , whole chromosomes [11] or even cases of the integration of almost complete genomes from bacterial endosymbionts into their eukaryotic hosts [12] have been described. Notable impacts of recently described horizontal transfers include key roles in land colonization by plants [13] , pigment production in spider mites through the acquisition of fungal carotenoid biosynthesis genes [14] and the emergence of plant diseases through transfers in fungi [15] . Despite these examples, the lack of specific evolutionary trends in reported cases of lateral gene transfer in eukaryotes has led to the view of ancient, sporadic and isolated events with relatively little global impact on eukaryotic kingdoms, rather than a more frequently and widely occurring phenomenon. The frequency and importance of eukaryote-to-eukaryote gene transfer may, however, be underestimated. Penicillium species are ubiquitous filamentous ascomycetes important to the biotechnology, biomedical and food industries. They commonly occur as food spoilage agents and opportunistic pathogens and are widely used as versatile cell factories. P. camemberti and P. roqueforti are used as starter cultures for cheeses. P. camemberti, used for the maturation of soft cheeses, such as Camembert, is the result of many selection programs aiming to improve the texture and colour of the conidia or physiological characteristics. P. camemberti has never been isolated from substrates other than dairy products. P. roqueforti is widespread in food and also occurs in silage and natural environments. It is used as a starter culture in the production of most blue-veined cheeses (including Roquefort, Gorgonzola, Stilton and Danish Blue) and its abilities to tolerate cold temperatures, low oxygen concentrations, alkaline and weak acid preservatives, make it a common spoilage agent in refrigerated stored foods, meat products, rye bread and silage [16] , [17] . To our knowledge, despite the importance of the filamentous fungi used in cheese making, no genome sequence has yet been published for any of these species. The availability of these first two genome sequences will therefore provide a useful resource for improving our knowledge of edible cheese moulds and for comparative genomics. Here we sequence and assemble the genomes of P. roqueforti and P. camemberti and compare them with two other available Penicillium genomes, those of the penicillin producer and food spoilage agent P. rubens , previously known as P. chrysogenum [18] , and of the Citrus pathogen P. digitatum [19] . We report a case of multiple, present-day horizontal transfers of a very large (over 500 kb) genomic island between several cheese fungi. This genomic island harbours about 250 genes, some of which are probably involved in competition with other microorganisms. Beyond the potential conceptual and applied implications of recurrent horizontal transfers occurring in food, this finding indicates that horizontal gene transfer (HGT) may be more widespread and important than previously thought in eukaryotes. 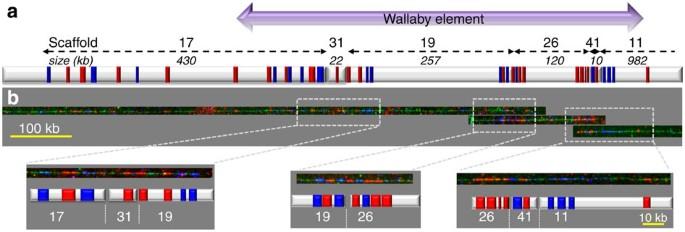Figure 1: Structural characterization of theWallabyregion inP. roquefortiFM164. (a)In silicogenomic Morse code for physical mapping, by molecular combing, of the six scaffolds bearing theWallabyelement (purple arrow). The numbers at the top indicate the scaffold names, with sizes in kilobases (kb) indicated below. (b) Visualization of the scaffolds mapped to theWallabylocus. Grey boxes show a higher magnification of scaffold junctions. Images are re-coloured based on fluorescence signal emission lengths. Green: YOYO-1 stained combed DNA fibre. Red: Probe detected with Alexa 594 conjugated antibodies. Blue: Probe detected using Alexa 394 and AMCA conjugated antibodies. Detection of a horizontally transferred genomic island The global characteristics and comparisons of the genomes of P. camemberti , P. roqueforti , P. rubens and P. digitatum are given in Table 1 . The genomes have similar sizes and number of genes, with the exception of P. digitatum , which has fewer genes than the other three genomes. This smaller number of genes is thought to be the result of a streamlining process affecting the genome of P. digitatum due to its specialized plant pathogenic lifestyle [19] . Assembly quality, as shown by the N50 metric and the number of scaffolds, is high for P. roqueforti and P. rubens . The initial in silico assembly for P. roqueforti has been experimentally validated and further improved (see below). The genome assemblies for P. camemberti and P. digitatum appear more fragmented. Table 1 Accession numbers and global characteristics of the Penicillium genomes compared in this study. Full size table Surprisingly, several scaffolds from P. roqueforti, P. camemberti and P. rubens had stretches of more than 5 kb displaying 100% identity in common ( Supplementary Fig. S1 ), whereas mean pairwise identity was, otherwise, only 85–90% between genomes. P. digitatum completely lacked these regions that were identical in the other Penicillium species. We investigated the nature of these shared sequences, by locating these regions accurately in the genome of P. roqueforti by improving assembly quality. The availability of a high-quality genome sequence in this clade will also improve the resolving power of comparative genome analysis in subsequent studies. For this purpose, we used a combination of polymerase chain reaction (PCR) and molecular combing, a powerful fluorescent in situ hybridization-based technique for the direct visualization of single-DNA molecules [20] , [21] . Molecular combing resulted in the successful mapping of scaffolds, including some separated by more than a 100 kb, onto single-DNA molecules, thus constituting a new means of improving or experimentally validating de novo genome assemblies ( Supplementary Fig. S2 ). It yielded an assembly in which 92% of the P. roqueforti genome was clustered into six super scaffolds of chromosomal sizes ( Supplementary Fig. S3 ). In the P. roqueforti FM164 strain, all the sequences found identical to both P. rubens and P. camemberti clustered together within a single 575 kb region accounting for 2% of the genome, which we called ‘ Wallaby ’ ( Figs 1 and 2 ). This region lies within a 7.8 Mb chromosome ( Supplementary Fig. S3 ). The genomes of additional strains of P. roqueforti were examined by SOLiD resequencing. Three lacked the entire Wallaby region, whereas the fourth carried the very same Wallaby sequence as FM164. These sequences were aligned for precise mapping of the Wallaby insertion point ( Fig. 3 ). Some of the regions flanking Wallaby could be characterized in P. rubens and P. camemberti and were found to share 85–90% identity in the three species. However, these sequences were located on other scaffolds than those carrying the Wallaby fragments in the two later species ( Fig. 2 ), indicating non-homologous locations of Wallaby between all three species. The possibility of misassembly yielding these different locations was excluded by the successful PCR amplification of fragments overlapping the edges of the identical sequences in the three genomes. Furthermore, rearrangement events appeared to have occurred after the transfers in all three species. Indeed, the Wallaby sequences of P. rubens and P. camemberti lacked various fragments present in P. roqueforti, and both contained a 86-kb fragment absent from P. roqueforti ( Fig. 2 ). Figure 1: Structural characterization of the Wallaby region in P. roqueforti FM164. ( a ) In silico genomic Morse code for physical mapping, by molecular combing, of the six scaffolds bearing the Wallaby element (purple arrow). The numbers at the top indicate the scaffold names, with sizes in kilobases (kb) indicated below. ( b ) Visualization of the scaffolds mapped to the Wallaby locus. Grey boxes show a higher magnification of scaffold junctions. Images are re-coloured based on fluorescence signal emission lengths. Green: YOYO-1 stained combed DNA fibre. Red: Probe detected with Alexa 594 conjugated antibodies. Blue: Probe detected using Alexa 394 and AMCA conjugated antibodies. 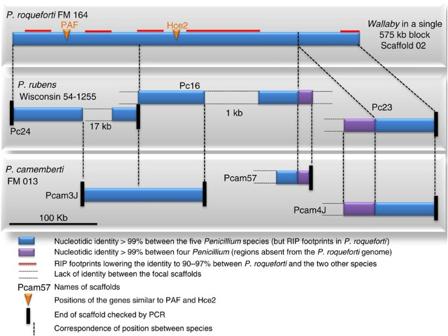Figure 2: Comparative genomic structure ofWallaby. The structure of the horizontally transferred genomic island is compared betweenP. roqueforti,P. rubensandP. camemberti. The sequence shown at the top corresponds to theWallabylocus inP. roquefortiFM164, that is, from positions 1,487,035 to 2,061,670. Full size image Figure 2: Comparative genomic structure of Wallaby. The structure of the horizontally transferred genomic island is compared between P. roqueforti , P. rubens and P. camemberti . The sequence shown at the top corresponds to the Wallaby locus in P. roqueforti FM164, that is, from positions 1,487,035 to 2,061,670. 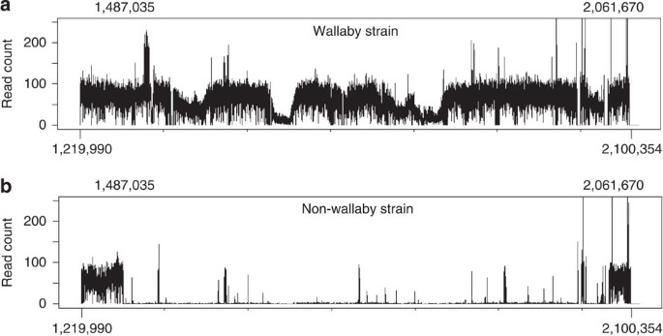Figure 3: Read mapping of the genomes of two additional strains against theWallabylocus of theP. roquefortiFM164. (a) A strain bearingWallabyisolated from cheese. (b) A strain not possessing Wallaby, isolated from an environment other than dairy products. This figure displays a count of the number of reads at each single base position. Thexaxis represents genomic coordinates. Theyaxis scale represents the number of reads counted for every position. Full size image Figure 3: Read mapping of the genomes of two additional strains against the Wallaby locus of the P. roqueforti FM164. ( a ) A strain bearing Wallaby isolated from cheese. ( b ) A strain not possessing Wallaby, isolated from an environment other than dairy products. This figure displays a count of the number of reads at each single base position. The x axis represents genomic coordinates. The y axis scale represents the number of reads counted for every position. Full size image Wallaby displayed little similarity to sequences from public databases, even those of the well-studied Aspergillus genus, the closest relative of Penicillium [18] . When Blast hits could be obtained, they matched fungal genomes ( Supplementary Fig. S4 ), indicating a fungal origin for Wallaby . A tetranucleotide composition analysis of Wallaby and its comparison with several fungal genomes revealed a nucleotide composition of Wallaby that seemed to be different from the rest of the genomes of P. rubens, P. camemberti and P. roqueforti, but still closer from these genomes than any other ( Table 2 and Supplementary Fig. S5 ). The nucleotide composition of Wallaby also differed from that of other available fungal genomes, but was nevertheless closest to Aspergillus and Penicillium strains, suggesting that the donor species lie within this clade ( Table 2 , Supplementary Fig. S5 ). Table 2 Pearson correlation coefficients for Z-score of tetranucleotide frequency. Full size table Overall, these results indicate that Wallaby has been recently and independently acquired, in at least some of these Penicillium species, via horizontal transfers. Other alternative explanations, such as introgression, can be excluded because of the non-homologous locations of the identical sequences in P. rubens and P. camemberti , precluding a parsimonious hybridization hypothesis. The perfect identity of the sequences also argues for very recent transfer events. No synonymous mutations were found in Wallaby , except for some repeat induced point (RIP) mutation footprints in P. roqueforti , indicating that the presence of Wallaby is not an ancestral character. Pairwise comparison of the genome-wide distribution of 100% identical sequences between P. roqueforti and the three other genomes revealed no long stretches of sequences identical in all three genomes other than those in Wallaby . The only variation within Wallaby thus corresponded to RIP mutation footprints in the P. roqueforti Wallaby region ( Fig. 2 ; Supplementary Fig. S6 ). In fungi, the RIP mechanism induces multiple C:G to T:A substitutions in repeated sequences during sex events [22] , [23] . As a consequence, sequence identity in Wallaby fragments with RIP footprints dropped to 90–97% between P. roqueforti and the other two Penicillium sequences, but this concerned exclusively RIP C:G to T:A substitutions. This is consistent with the occurrence of RIP after the transfer event in P. roqueforti . The region flanking Wallaby in P. roqueforti may be a hotspot for DNA insertions, as other unrelated fragments appear to be inserted at this locus in other Penicillium genomes ( Fig. 4 ). However, no footprints of duplication or transposable elements were found around the Wallaby insertion points for which flanking regions could be identified. 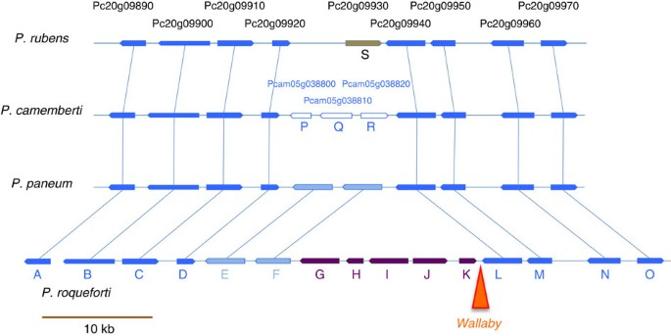Figure 4: Schematic representation of the flanking regions ofWallabyinP. roqueforticompared with homologous regions in otherPenicilliumspecies. Predicted genes are indicated, and those for which homology could be detected in this region in other species are linked and blue. White predicted genes have no detectable similarity to sequences in this region from other species.WallabyinP. roquefortiis indicated by a red triangle. TheP. camembertiandP. rubens Wallabyregions are fragmented and located in non-homologous regions and are therefore not shown on this figure.P. paneumdoes not carryWallaby. Figure 4: Schematic representation of the flanking regions of Wallaby in P. roqueforti compared with homologous regions in other Penicillium species. Predicted genes are indicated, and those for which homology could be detected in this region in other species are linked and blue. White predicted genes have no detectable similarity to sequences in this region from other species. Wallaby in P. roqueforti is indicated by a red triangle. The P. camemberti and P. rubens Wallaby regions are fragmented and located in non-homologous regions and are therefore not shown on this figure. P. paneum does not carry Wallaby. Full size image Wallaby transfer to several other species The presence of Wallaby was further investigated in 441 strains by PCR amplification with Wallaby- specific primers, designed from single-copy putative coding sequences, each amplifying 1 kb ( Supplementary Table S1 ). We carried out an exhaustive screening of all the terverticillate Penicillium species, the clade to which P. roqueforti, P. camemberti and P. rubens belong, from the public collection of the MNHN, as well as subsets of additional collections, including strains isolated from various ecological niches, corresponding to 51 morphospecies ( Fig. 5 , Supplementary Tables S2–S4 ). Amplicons were obtained for all P. camemberti strains and a fraction of the strains from P. roqueforti and from the P. chrysogenum — P. rubens clade. The amplicons were sequenced and all were identical to Wallaby sequences. The lack of non-synonymous substitutions in all these species further indicates that the presence of Wallaby is not an ancestral character. Several strains from species closely related to P. camemberti and present in dairy environments or occurring as food contaminants, such as P. caseifulvum, P. biforme, P. fuscoglaucum, P. palitans, P. solitum, P. nordicum and P. polonicum, for example, also gave amplicons ( Fig. 5 ; Supplementary Tables S2 and S3 ). No amplicons were obtained from P. roqueforti s trains isolated from other environmental niches or from Penicillium species not associated with cheese environments (for example, P. carneum, P. expansum, P. cavernicola ), other than P. chrysogenum s. l., that is, the species complex encompassing both P. chrysogenum and P. rubens ( Fig. 5 ; Supplementary Tables S2 and S3 ). 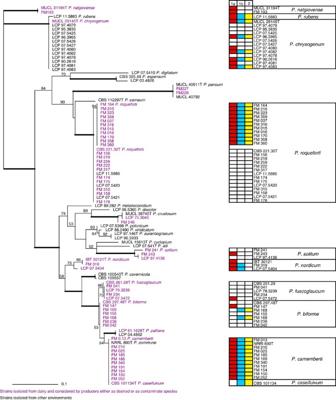Figure 5: Gene genealogy for thePenicilliumstrains screened by PCR for the presence ofWallabyand for which DNA sequences of the markers could be obtained. Penicilliumspecies associated with the cheese environment are indicated in purple. Colours in the pseudotable indicate positive amplification for the three primer pairs (red, blue and yellow, respectively) for single-copy predicted genes inWallaby. Figure 5: Gene genealogy for the Penicillium strains screened by PCR for the presence of Wallaby and for which DNA sequences of the markers could be obtained. Penicillium species associated with the cheese environment are indicated in purple. Colours in the pseudotable indicate positive amplification for the three primer pairs (red, blue and yellow, respectively) for single-copy predicted genes in Wallaby . Full size image Transferred region is potentially involved in competition In P. roqueforti, Wallaby was predicted to contain 248 genes, 149 of which were covered by expressed sequence tags. No expanded gene families were detected within Wallaby. Few genes could be annotated ( Table 3 and see Supplementary Fig. S7 for the gene ontologies recovered) and Fisher’s exact tests indicated no significant enrichment of any particular function. Interestingly, some of the annotated genes were predicted to be involved in the regulation of conidiation (spore production) or in antimicrobial activities, suggesting functional advantages for Wallaby -bearing strains associated with competition in the cheese, which contain many other microorganisms. Table 3 Putative functions of the genes located in the flanking regions of Wallaby in P. roqueforti . Full size table In particular, among expressed genes within Wallaby , afp (gene ID: ProqFM164S02.2755) encodes a protein identical to PAF (Penicillium antifungal protein), with 100% nucleotide sequence identity to the paf gene of P. rubens ; PAF has been experimentally shown to be cytotoxic to fungi [24] and to regulate spore production [25] . Another expressed protein with putative antimicrobial activities, ProqFM164S02g002866 (gene ID: ProqFM164S02.2870), matched to Hce2 [26] , which has an Ecp2 domain—originally identified as a virulence factor in Cladosporium fulvum —fused to a GH18 chitinase domain very similar to the α subunit of the yeast killer toxin zymocin from the dairy yeast Kluyveromyces lactis [27] . Hce2 proteins with such an architecture are thought to play a role in antagonistic interactions with other microorganisms [26] . The sequencing of the first two genomes of food Penicillium strains will provide an invaluable resource for comparative genomics of fungi, nicely complementing the 1,000 fungal genomes project and the JGI fungal genome initiative, in which no Penicillium from the food environment is being sequenced. We also report here the development and application of a methodology for improving and validating genome assemblies based on an original single-DNA molecule technology, molecular combing. Improving genome assembly, notably by the use of physical maps, has been largely advocated [28] , [29] , and is even deemed crucial for comparative genomics [30] . Our data indicate that food Penicillium strains contain regions, grouped at a single location and called Wallaby in P. roqueforti, that have very recently undergone multiple horizontal transfers. Several lines of evidence support the acquisition of Wallaby by horizontal transfer and rule out alternative hypotheses. First, an ancestral presence of Wallaby is refuted by the complete identity (except for RIP mutation footprints in some fragments in P. roqueforti ), even in noncoding regions, over more than 500 kb, between distant species with genome sequence identities otherwise of about 90%, and by the absence of Wallaby from all fungal species other than those in which it is identical. Furthermore, the non-homologous locations rule out introgression and the presence of Wallaby almost exclusively in species from the food environment and the different nucleotide composition of Wallaby from the rest of the recipient genomes provide further support for horizontal transfer. The nucleotide composition of Wallaby suggests that the donor species may belong to the Aspergillus or Penicillium clade. The function of one of the genes contained in Wallaby, experimentally demonstrated in P. rubens [24] , suggests that it may confer adaptation associated with competition with other microorganisms. The occurrence of gene transfers in fungi has been reported before [1] , [11] , [31] , [32] , but this case of HGT is exceptional in several ways. The Wallaby genomic islands are unusually large, covering 2% of the host genomes. Furthermore, these sequences were found to be 100% identical in the species screened, with the exception of the RIP mutation footprints in P. roqueforti . The complete identity of the transferred sequences and the lack of corresponding sequences in databases prevent phylogenetic reconstruction of the history of transfers. However, we can hypothesize that the original donor had a complete island in a single block, as in P. roqueforti, and that this block was then transferred to other acceptor genomes, in which it was fragmented and may then have been transferred to other species. Some of the P. rubens scaffolds containing Wallaby, Pc23 and Pc24 have already been shown to be absent from P. digitatum [19] . This study also showed that several fragments of these scaffolds matched other dispersed elements in the genome of P. rubens , with an identity of about 90%. It has been suggested that this level of similarity indicated gene family expansion rather than horizontal transfer [19] . Our analysis of additional sequenced genomes revealed that these dispersed elements were specific to P. rubens and that horizontal transfers occurred in addition to possible gene family expansions. The widespread occurrence of Wallaby in cheese species, including species never found in other environments, such as P. camemberti, together with the identity of the sequences indicate that these transfers occurred in cheese and were, therefore, very recently promoted by human activities. Such horizontal transfers may be facilitated by the ability of fungi to form anastomoses—somatic fusions between mycelia known to occur in Penicillium species [33] , [34] —and may facilitate the transfer of whole chromosomes in fungi grown in laboratory environment [11] . Functions brought by the transferred material may, therefore, be beneficial in the food environment, as suggested by the functions identified in Wallaby, involved in antagonistic interactions with other microorganisms [26] . This study provides strong support for the view that horizontal transfers of large genomic regions play an important role in fungal adaptation to new environments [35] , [36] , including those created by humans. The example reported here is, however, unique to date among transfers, in terms of the size of the region transferred, its total identity between species and the number of species involved. Horizontal gene transfer in fungi may be beneficial, particularly in cheese making strains or wine yeasts, in which large transfers of genes promoting fermentation have been detected [1] . The data presented here, particularly when considered in the light of the growing list of reports of horizontal gene transfer between eukaryotes, suggest that this phenomenon may occur frequently and may have a wider impact than previously thought, as already advocated [3] , [5] . We foresee major implications for the management of pathogen species in the face of current changes, including globalization, which may bring previously isolated species into contact. Rapid evolution by horizontal gene transfer may also have a major impact through the emergence of new diseases caused by fungi acquiring new virulence genes horizontally [7] , [10] , [11] , [15] , [37] . Furthermore, in itself, this finding indicates that horizontal gene transfer can occur within the food chain. The frequency of this phenomenon should be investigated more thoroughly, as it may have a potential impact on food, agricultural and biotechnological practices. DNA extraction and genome sequencing DNA was extracted with the cetyltrimethylammonium bromide (CTAB) extraction procedure [38] , [39] , [40] . Mycelium (10 g) was recovered from ~10 Petri dishes and frozen with liquid nitrogen in a mortar. The mycelium was ground to a powder and 10 ml of 2 × CTAB buffer was added. The frozen mixture was left to thaw, quickly transferred to a 50 ml Corning tube and placed in a 65 °C water bath for 30 min. One volume of chloroform/isoamyl alcohol was then added and the solution was mixed thoroughly to form a complete emulsion. After a centrifugation step of 10 min at 4,000 g , the top aqueous phase (above the chloroform phase and mycelium fragments) was transferred into a new 50 ml tube; 1/5 volume of 5% CTAB solution was added and the chloroform/isoamyl alcohol extraction step was performed again, except for the addition of the 5% CTAB solution at the end. The top aqueous phase was gently mixed with an equal volume of CTAB precipitation buffer and the resulting solution was incubated for 1 h at room temperature to form a precipitate. After 10 min of centrifugation at 4,000 g , the supernatant was discarded and the precipitate dissolved into 2 ml of high-salt TE (pH 8.0) [10 mM tris(hydroxymethyl)aminomethane (TRIS), 1 mM ethylenediaminetetraacetic acid (EDTA) and 1 M NaCl]. Nucleic acids were precipitated with 4 ml of cold ethanol, pelleted in Corex tubes and washed with 4 ml of 70% ethanol. The nucleic acid pellet was left to dry. The pellet was resuspended into 4 ml of TE (pH 8.0) (10 mM TRIS, 1 mM EDTA). Nuclear DNA was purified and excess mitochondrial DNA was eliminated by centrifugation on a caesium gradient with 4′,6-diamidino-2-phenylindole (DAPI) [41] . We added 1.15 g solid caesium chloride and 4 μl of DAPI solution (1 mg ml −1 ) per ml of DNA solution (final density: 1.65 g ml −1 ). The DNA/CsCl/DAPI solution was centrifuged in a Quick-Seal centrifuge tube (part #342412, Beckman, Palo Alto, USA) at 50,000 r.p.m., for 12–15 h, in a Beckman VTi65 vertical rotor. Two bands of DNA were visible under UV light. The lower band (that is, nuclear DNA, the upper band corresponding to mitochondrial DNA) was collected with a syringe (1.2 × 40 mm needle); DAPI was extracted with isoamyl alcohol saturated with CsCl (1.15 g ml −1 ) and the DNA solution was dialyzed for 4 days against 10 mM TRIS, 1 mM EDTA (pH 8.0) with twice-daily replacement of the dialysis solution. Sequencing and annotation Penicillium camemberti FM 013 and P. roqueforti FM164 were sequenced by Genoscope (Evry, France), via the 454 sequencing of an 8 kb mate pair library (793786 and 661034 cleaned read pairs, respectively) combined with Illumina Solexa sequencing (34126183 and 34253031 76 nt single-end reads, respectively). Assembly was performed with SOAPdenovo v1.05 and velvet v1.1.04 (ref. 42 ). SOAPdenovo was run (kmer values 43–67) to generate contigs. Velvet was then run with combined raw reads and SOAPdenovo contigs (parameters ‘-cov_cutoff 5 -min_contig_lgth 100 -max_divergence 0.05 -long_mult_cutoff 1 -exp_cov auto’). The range of kmer values for Velvet was 41–57. The short-reads assembly with the maximum N50 value was used as input for the scaffolding process (SOAPprepare and SOAPdenovo). For P. roqueforti , maximum N50 values were obtained with a kmer value of 37 and a minimum of six links between contigs (parameter (default=5) pair_num_cutoff=6). For P. camemberti , a kmer value of 27 and a minimum of 14 links gave the highest N50 value. Gene models were predicted with EuGene [43] , [44] , a highly integrative eukaryotic protein-coding gene prediction platform. This gene predictor requires training: a data set of 442 curated gene models was built and split into three homogeneous, independent data sets. The first was used for training, the second for parameter optimization and the third for performance evaluation. We used for genome annotation 13,878 ESTs, resulting from the assembly of 780,051 cDNA sequences from P. roqueforti , together with the Swiss Protein database (February 2011), the proteomes of Saccharomyces cerevisiae and P. chrysogenum Wisconsin 54-1255, a database of all Eurotiales proteins in GenBank HG765102–HG778979 (February 2011). Transposable elements were identified with REPET [45] . InterPro was used to identify protein domains and families. The P. roqueforti FM164 draft genome was assembled before molecular combing into 73 scaffolds of over 2 kb, spanning 28 Mb. The P. camemberti FM 013 draft genome spans 34 Mb, assembled into 140 scaffolds of over 2 kb. Fungal isolates and single-spore isolation We used 441 isolates in total ( Supplementary Tables S2–S4 ). The 124 isolates provided by producers of starter cultures and cheeses were labelled FM and their origins are confidential. All were isolated from the cheese environment and belong to four distinct ascomycete genera: Penicillium, Fusarium, Scopulariopsis and Sporendonema [46] . We analysed all 241 terverticillate Penicillium strains from the public collection of the MNHN, and some Eupenicillium species. We also analysed the LUBEM-Brest collection encompassing 76 P. roqueforti isolates, labelled with an F. These isolates were obtained from blue cheeses from 14 countries. The numbers after the ‘F’ correspond to individual cheeses. For the 39 cheeses, morphologically different strains were treated as different strains, labelled by a number following that identifying the cheese (for example, F17.1 and F17.2 are two strains from cheese 17). Single-spore isolation was systematically performed by the dilution method, after growth for 3–5 days at 25 °C on malt agar. The ‘F’ strains were also obtained by spore dilution. DNA extraction for PCR amplification Genomic DNA was extracted from fresh mycelium of the isolates listed in Supplementary Tables S2–S4 . Mycelium was obtained after 3–5 days on malt agar for Penicillium , Scopulariopsis and Fusarium strains and on a confidential medium provided by starter producers for Sporendonema casei . The Qiagen DNeasy Plant Mini Kit (Qiagen Crawley, UK) was used for DNA extraction. PCR amplification and sequencing of amplicons PCR was performed in a volume of 50 μl, containing 25 μl template DNA, 1.25 U AmpliTaq DNA polymerase (Roche Molecular Systems, Branchburg, NJ, USA), 5 μl 10 × Taq DNA polymerase buffer, 5 μl 50% glycerol, 2 μl 5 mM dNTPs, 2 μl of each 10 μM primer and 50–100 ng template DNA. Strains were identified with the 5′ end of the β-tubulin gene, with primers Bt2a/Bt2b (ref. 47 ). The three primer pairs designed to detect Wallaby are shown in Supplementary Table S1 . DNA fragments PC4 and PC13 (ref. 48 ) were used for the phylogenetic analysis. Amplifications were performed with 30 cycles of 30 s at 95 °C, 30 s at 58 °C for the three Wallaby primers, amplifying 1 kb each, and 2 min at 72 °C. For microsatellite loci, the thermal regime was 35 cycles of 30 s at 94 °C, 30 s at 50 °C and 30 s at 72 °C. All PCR programs had a final 5 min extension step at 72 °C. PCR products were purified and sequenced by Genoscope (Évry, France). Protoplast preparation for molecular combing A P. roqueforti conidial suspension was plated on M3 medium (0.25 g l −1 KH 2 PO 4 , 0.3 g l −1 K 2 HPO 4 , 0.25 g l −1 MgSO 4 , 0.5 g l −1 urea, 0.05 mg l −1 thiamine, 0.25 μg l −1 biotin, 2.5 mg l −1 citric acid, 2.5 mg l −1 ZnSO 4 , 0.5 mg l −1 CuSO 4 , 125 μg l −1 MnSO 4 , 25 μg l −1 boric acid, 25 μg l −1 sodium molybdate, 25 μg l −1 iron alum, 5 g l −1 glucose, 25 mg l −1 chloramphenicol in seven Petri dishes and incubated 4 days at 25 °C. Conidia were harvested and resuspended in 20 ml M3 medium. Two 50 ml M3 medium liquid cultures were inoculated with the conidial suspension. Germination occurred after 18 h of incubation at 25 °C, with shaking at 90 r.p.m. The germinating conidia were harvested by centrifugation (10 min, 2,640 g ). Dried mycelium (1 g) was suspended in the protoplast isolation solution (400 mg Filtrozym (Laffort), 20 mg bovine serum albumin in 10 ml of TRF1 solution (1.2 M MgSO 4 , 10 mM orthophosphate, pH 5.8). The suspension was incubated at 30 °C for 120–150 min, with shaking at 90 r.p.m. Once the cell walls had been lysed, we transferred the 10 ml suspension to a 30 ml glass tube and overlaid it with 10 ml TRF2 (0.6 M sorbitol, 100 mM Tris-HCl pH 7.5). After centrifugation for 10 min at 2869 g at room temperature, the protoplasts formed a layer at the interface. The protoplast layer was removed and washed with an equivalent volume of TRF3 (1 M sorbitol, 10 mM Tris-HCl pH 7.5), by centrifugation at 2,640 × g for 10 min. The protoplast pellet was suspended in 1 ml TRF4 solution (1 M sorbitol, 10 mM Tris-HCl pH 7.5, 10 mM CaCl 2 ). Molecular combing Molecular combing and suitable hybridization, detection and scanning procedures were performed according to conventional combing procedures [49] , [50] . Molecular combing experiments involve embedding cells into an agarose plug, releasing DNA into solution by digesting this plug, stretching the DNA on a coverslip with a molecular combing system and performing fluorescent in situ hybridization experiments on the combed DNA. Briefly, P. roqueforti FM164 protoplast prepared as described above were embedded in agarose plugs. Protoplasts were lysed overnight by incubation in a 1% sarkosyl, proteinase K (2 mg ml −1 ) in 0.5 M EDTA pH 8.0 at 50 °C. Agarose plugs were then washed in 10 mM Tris, 1 mM EDTA pH 8.0. Genomic DNA was stained by incubating the plug in a 40 mM Tris, 2mM EDTA, 3 μl YoYo-1 solution for 1 h. The combing solution containing the genomic DNA was obtained by melting agarose at 68 °C for 20 min and subsequently digesting agarose molecules using β-agarase (42 °C, overnight). DNA fibres were combed on combicoverslips using the molecular combing system (both from Genomic Vision, France). The PCR amplicons for probe production were purified and used directly as templates for the labelling reaction, rather than after subcloning (primer sequences available on request). Probes were labelled by random priming and revealed using Alexa 594 (red), Alexa 350/AMCA (blue) conjugated antibody sandwiches. The combed DNA was counterstained after the fluorochrome detection step, by incubating the coverslip in 30 μl of a 1:1,000 YoYo-1 solution in milli-Q water for 30 s and then washing three times, for three minutes each, in milli-Q water. Genomic Morse codes (GMC) were designed at the extremities of scaffolds. A GMC is a signal generated by a set of specifically designed probes. A GMC consists of an alternating series of dots, dashes (probes) and gaps (region between two probes) of different sizes and colours, designed to generate an unambiguous pattern at a specific locus, thus physically mapping the region [51] . GMCs at the extremities of scaffolds generate unambiguous patterns making it possible to locate and orient scaffolds accurately on single-stretch DNA molecules, by combining two Morse codes in cases of neighbouring scaffolds. In the case of distant scaffolds, the distance separating the scaffolds is measured based on the distance separating the two genomic Morse codes ( Supplementary Fig. S2 ). Phylogenetic analysis Genealogical relationships were inferred using the flanking regions of the two microsatellite loci PC4 and PC13 (classical loci like the β-tubulin gene are not variable enough). Sequences were manually aligned, with BioEdit [52] . Independent phylogenetic trees were built with TreeFinder [53] under a maximum likelihood framework. A nucleotide substitution model (GTR+G) was inferred with jmodeltest [54] . As the two topologies were congruent, we concatenated the data sets to obtain a single phylogenetic tree based on 363 bp. Branch support was determined from a bootstrap analysis of 1,000 re-sampled data sets. RIP mutation analysis Using fragments of the Wallaby sequences of P. roqueforti FM164, P. camemberti FM 013 and P. rubens Wisconsin 54-1,255, we searched for RIP-like footprints [55] . Multiple sequence alignments were built, using ClustalW with default settings [56] . RIP mutation-like footprints were sought with RIPCAL software [57] ( Supplementary Fig. S6 ). Tetranucleotide composition Correlations between Z -scores of tetranucleotide composition were assessed using jspecies version 1.2.1 61 . Accession codes: Genome sequence data for P. roqueforti have been deposited in the GenBank nucleotide core database under the accession codes HG792015 to HG792062 . Genome sequence data for P. camemberti have been deposited in the GenBank nucleotide core database under the accession codes HG793134 to HG793313 . The EST sequence data of P. roqueforti used for genome annotation have been deposited in the EMBL-EBI database under the accession codes HAAZ01000001 - HAAZ01013080 . How to cite this article: Cheeseman, K. et al. Multiple recent horizontal transfers of a large genomic region in cheese making fungi. Nat. Commun. 5:2876 doi: 10.1038/ncomms3876 (2014).